The Ufm1-activating enzyme Uba5 is indispensable for erythroid differentiation in mice Post-translational protein modifications are systems designed to expand restricted genomic information through functional conversion of target molecules. Ubiquitin-like post-translational modifiers regulate numerous cellular events through their covalent linkages to target protein(s) by an enzymatic cascade analogous to ubiquitylation consisting of E1 (activating), E2 (conjugating) and E3 (ligating) enzymes. In this study, we report the essential role of Uba5, a specific activating enzyme for the ubiquitin-like modifier, Ufm1, in erythroid development. Mice lacking Uba5 exhibited severe anaemia, followed by death in utero . Although Uba5 was dispensable for the production of erythropoietin, its genetic loss led to impaired development of megakaryocyte and erythroid progenitors from common myeloid progenitors. Intriguingly, transgenic expression of Uba5 in the erythroid lineage rescued the Uba5- deficient embryos from anaemia and prolonged their survival, demonstrating the importance of Uba5 in cell-autonomous erythroid differentiation. Our results suggest that one of the ubiquitin-like protein modification systems, the Ufm1 system, is involved in the regulation of haematopoiesis. Emerging evidence during the past decade has highlighted the importance of ubiquitin and ubiquitin-like proteins (UBLs), which conjugate with target molecules through an elaborate enzymatic reaction consisting of E1, E2 and E3 (refs 1 , 2 , 3 , 4 ). In the initial step, ubiquitin is activated by a ubiquitin-activating enzyme, E1, which forms a high-energy thioester bond with ubiquitin by means of adenylation in an ATP-dependent manner. In the second step, the E1-activated ubiquitin is transferred to a ubiquitin-conjugating enzyme, E2, using a thioester linkage. In some cases, an E2 can directly transfer the ubiquitin to substrate proteins through an isopeptide linkage; however, E2s mostly require the participation of a ubiquitin-ligating enzyme, E3, to achieve a substrate-specific ubiquitylation reaction in the cells. Although the covalent modification of cellular proteins with ubiquitin mainly mediates selective protein turnover, modification of intracellular proteins by the UBLs regulates protein localization, protein–protein or protein–DNA interactions and/or biochemical activities. Therefore, these modifications serve various physiological events, including cell survival, differentiation and death [3] , [4] . Haematopoiesis is a complex process orchestrated by specific transcription factors and cytokines that support the self-renewal, differentiation and survival of haematopoietic progenitors at different stages of maturation, and defects in these processes often lead to pathological conditions such as leukaemia and myelodysplastic syndrome [5] , [6] . Among UBLs, SUMO regulates erythroid differentiation through sumoylation of GATA1, which is crucial for the control of production of erythrocytes, platelets, mast cells and eosinophils [7] , [8] . Two other UBLs, Atg8 and Atg12, which are essential for autophagy, also contribute to mitochondrial elimination by autophagy in developing erythrocytes [9] , [10] , [11] . Apart from SUMO and autophagy-related UBLs, however, little is known about the biological significance of other UBLs in the complex process of haematopoiesis. Ubiquitin-fold modifier 1 (Ufm1) is a recently identified protein modifier [12] . Ufm1 is synthesized in a precursor form and cleaved at the carboxy terminus by specific proteases such as UfSPs [13] . Thereafter, an E1-like enzyme, Uba5, activates the mature Ufm1, forming a high-energy thioester bond. The activated Ufm1 is then transferred to an E2-like enzyme, Ufc1, through a similar thioester linkage [12] . Finally, Ufm1 is covalently conjugated with functionally as-yet-unknown cellular proteins via Ufl1 (E3-ligating enzyme) [14] . The conjugates are cleaved by UfSPs, implying the reversibility of the Ufm1-conjugating system ('ufmylation') [13] , [14] . Because all molecules (that is, Ufm1, Uba5, Ufc1, Ufl1 and UfSPs) involved in ufmylation are conserved in metazoa and plants, but not in yeast, the potential roles in various multicellular organisms are of special interest. However, the physiological functions of the Ufm1 system are completely unknown. In this study, we provided evidence that Uba5 is a specific activating enzyme for a ubiquitin-like modifier, Ufm1, and generated a Uba5 -deficient mouse model. Remarkably, these mice died in utero because of severe anaemia associated with defective differentiation of both megakaryocytes and erythrocytes. These defects were rescued by Uba5 expression in the erythroid and megakaryocytic progenitors, implying cell-autonomous impairment of erythropoiesis in Uba5 −/− mice. Our results suggest that the Ufm1 system has an essential role in erythroid differentiation. Uba5 is a specific activating enzyme for Ufm1 Eight activating enzymes for ubiquitylation and UBL modification can be identified in the human genome by computer-assisted homology analysis ( Supplementary Table S1 ) (ref. 4 ). Although most activating enzymes activate single targets among the UBLs, some E1-like enzymes can activate two distinct UBLs [15] , [16] , [17] . It was recently reported that Uba5 also activates SUMO2, in contrast to the original claim that addressed the specificity for Ufm1 (ref. 18 ). Thus, we first attempted to clarify this problematic issue. To determine whether Uba5 can activate proteins other than Ufm1, we used an Uba5-mutant in which the active site, cysteine (Cys250), was substituted with serine (termed Uba5 C250S ). When the active-site cysteine residue within E1 and E1-like enzymes is replaced with serine, an O -ester bond is formed instead of a thioester bond with its respective modifier proteins, and the intermediates become stable even under reducing conditions [12] . We expressed a FLAG-tagged Uba5 C250S (FLAG-Uba5 C250S ) together with each green fluorescent protein (GFP)-tagged UBL in HEK293T cells, and then the cell lysate was immunoprecipitated with anti-FLAG antibody, followed by immunoblot analysis. An intermediate between FLAG-Uba5 C250S and GFP-Ufm1, but not other GFP-UBLs, was clearly recognized ( Supplementary Fig. S1a ). Moreover, loss of Uba5 had no apparent effect on UBL conjugations except for Ufm1 conjugation ( Supplementary Fig. S1b ). These results suggest that Uba5 is a specific E1 enzyme for Ufm1. Generation of Uba5 knockout mice To investigate the in vivo functions of the Ufm1 system in mammals, we generated the Uba5 knockout mouse line. The mouse Uba5 gene is encoded by 12 exons that span a 15-kb genomic DNA sequence. The active-site cysteine residue, which is essential for the activation of Ufm1, is encoded by exon 7. Thus, the targeting vector was designed to substitute this exon with a neomycin resistance gene cassette ( Supplementary Fig. S2a ). Disruption of Uba5 was confirmed by the absence of both Uba5 transcript and protein in Uba5 -homozygous-null ( Uba5 −/− ) mouse embryonic fibroblasts (MEFs; Supplementary Fig. S2b,c ). We also tested the loss of Uba5 activity by examining Ufm1 conjugation in MEFs and confirmed the loss of Ufm1 conjugates with some cellular targets (for example, 39- and 51-kDa proteins; Supplementary Fig. S2c ). Loss of Uba5 leads to death in utero due to severe anaemia All Uba5 −/− mice from Uba5 +/− intercrosses died in utero , whereas Uba5 -heterozygous ( Uba5 +/− ) mice were born healthy and fertile without any noticeable pathological phenotype for at least 2 years. These results indicate that the complete loss of Uba5 is embryonically lethal. 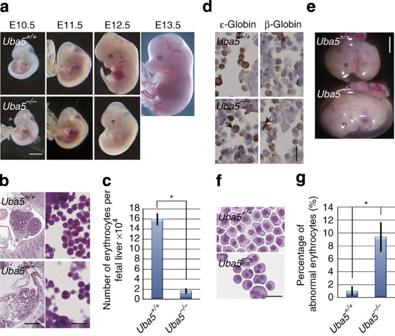Figure 1: Loss ofUba5leads to deathin uterobecause of severe anaemia. (a) Morphological examination ofUba5−/−mice embryos. Representative photographs ofUba5+/+andUba5−/−embryos at various developmental stages.Uba5−/−embryo at E12.5 exhibited severe anaemia. Scale bar, 2 mm. (b) Haematoxylin and eosin staining of fetal liver sections ofUba5+/+andUba5−/−mice at E11.5. Scale bars: left panel, 1 mm; right panel, 20 μm. (c) Number of erythrocytes in fetal livers ofUba5+/+andUba5−/−mice at E11.5. (d) Immunohistochemistry of fetal liver sections ofUba5+/+andUba5−/−embryos at E11.5 with anti-ɛ-globin and anti-β-globin antibodies. Arrows: abnormal multinucleated erythrocytes. Scale bar, 20 μm. (e) Representative photographs ofUba5+/+andUba5−/−embryos at E11.5. The circulating erythrocyte volume is reduced in the yolk sac ofUba5−/−embryos. Scale bar, 2 mm. (f) Wright–Giemsa staining of peripheral blood cytospin cells prepared from the indicated genotypes at E11.5. Scale bar, 20 μm. (g) Percentage of abnormal erythrocytes shown inf. Bar graphs incandgshow the mean±s.d. values of five mice from each group. Statistical analysis was carried out using the unpairedt-test. *P<0.05 (Welch test). Analysis of Uba5 −/− embryos at different developmental stages showed that the majority of embryos died between 12.5 and 13.5 embryonic days (E) after gestation ( Table 1 ). The Uba5 −/− embryos appeared paler and smaller than their wild-type littermates ( Fig. 1a ). The most obvious phenotype was severe fetal anaemia. Table 1 Genotype analysis of Uba5 heterozygous intercross progeny. Full size table Figure 1: Loss of Uba5 leads to death in utero because of severe anaemia. ( a ) Morphological examination of Uba5 −/− mice embryos. Representative photographs of Uba5 +/+ and Uba5 −/− embryos at various developmental stages. Uba5 −/− embryo at E12.5 exhibited severe anaemia. Scale bar, 2 mm. ( b ) Haematoxylin and eosin staining of fetal liver sections of Uba5 +/+ and Uba5 −/− mice at E11.5. Scale bars: left panel, 1 mm; right panel, 20 μm. ( c ) Number of erythrocytes in fetal livers of Uba5 +/+ and Uba5 −/− mice at E11.5. ( d ) Immunohistochemistry of fetal liver sections of Uba5 +/+ and Uba5 −/− embryos at E11.5 with anti-ɛ-globin and anti-β-globin antibodies. Arrows: abnormal multinucleated erythrocytes. Scale bar, 20 μm. ( e ) Representative photographs of Uba5 +/+ and Uba5 −/− embryos at E11.5. The circulating erythrocyte volume is reduced in the yolk sac of Uba5 −/− embryos. Scale bar, 2 mm. ( f ) Wright–Giemsa staining of peripheral blood cytospin cells prepared from the indicated genotypes at E11.5. Scale bar, 20 μm. ( g ) Percentage of abnormal erythrocytes shown in f . Bar graphs in c and g show the mean±s.d. values of five mice from each group. Statistical analysis was carried out using the unpaired t -test. * P <0.05 (Welch test). Full size image In mouse embryos, primitive erythropoiesis, which is characterized by the production of nucleated erythrocytes, is initiated in the yolk sac blood island at E7.0. On the other hand, definitive erythropoiesis starts around E11.5 in fetal livers, in which massive amounts of enucleated erythrocytes are produced from erythroblasts [19] . Haematopoietic stem cells in fetal livers continuously replenish erythroid progenitors for the production of erythrocytes to support embryos during late gestation [19] . At E11.5, the total number of nucleated erythrocytes in Uba5- deficient liver was markedly lower than in the corresponding tissue of wild-type mice ( Fig. 1b and c ). Occasionally, we observed multinucleated erythrocytes in the mutant fetal livers ( Fig. 1b ). These abnormal erythrocytes comprised ɛ-globin-positive primitive and β-globin-positive definitive erythrocytes ( Fig. 1d ), implicating impairment of both primitive and definitive erythropoiesis in Uba5 -knockout embryos. Indeed, we noticed reduced circulating erythrocytes in the yolk sac ( Fig. 1e ) and abnormal multinucleated erythrocytes in peripheral blood ( Fig. 1f,g ). Uba5 is essential for the development of erythroid lineage Haematopoietic progenitor cells can be accurately classified on the basis of their developmental potential, as schematically represented in Supplementary Figure S3a . Each type of erythroblast can be distinguished by examining the expression profiles of certain surface proteins such as CD71 and Ter119 (ref. 20 ; Supplementary Fig. S3b ). At E11.5, although Ter119 med CD71 high proerythroblasts and Ter119 high CD71 high basophilic erythroblasts were present in wild-type fetal livers, the numbers of both types of cells were diminished in Uba5 −/− fetal livers (10.0±1.2% versus 4.2±3.2% and 23.6±1.6% versus 1.0±0.6%, respectively, n =3, P <0.05, Fig. 2a ). Next, we compared erythroid colony-forming units (CFU-Es) and more immature erythroid burst-forming units (BFU-Es) in wild-type and Uba5 −/− fetal livers at E11.5. Both types of colonies were formed even in the absence of Uba5 . However, the number of Uba5 −/− CFU-Es ( Fig. 2b ) and BFU-Es ( Fig. 2c ) was significantly lower than in wild-type CFU-Es and BFU-Es (58.9% and 33.0%, respectively, P< 0.05), suggesting reduced numbers of erythroid progenitors. Furthermore, the colony formation assay for megakaryocyte (CFU-Megs) indicated that cells derived from Uba5 -knockout fetal livers had a reduced ability to form colonies (see Fig. 4d). These results indicate that loss of Uba5 is associated with defective differentiation of both megakaryocytes aned erythrocytes. 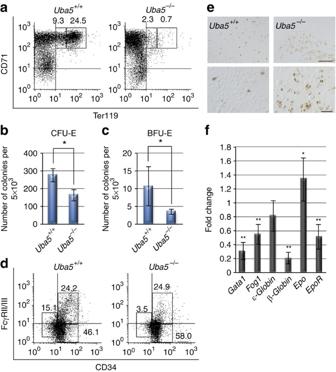Figure 2:Uba5is indispensable for the development of erythroid cells. (a) Representative FACS analysis. Mouse fetal liver cells were freshly isolated from E11.5 embryos and labelled with a FITC-conjugated anti-CD71 monoclonal antibody and PE-conjugated anti-Ter119 antibody.Left gate: proerythroblast population (Ter119medCD71high),right gate: basoerythroblast population (Ter119highCD71high). Axes mean log10fluorescent intensity. (b) Quantification of erythroid colony-forming units (CFU-Es) and (c) erythroid burst-forming units (BFU-Es). Colony assays were carried out with cells prepared from fetal liver at E11.5.Uba5deletion was associated with decreased erythroid progenitor activity. Data are means±s.d. of five mice from each group. Statistical analysis was performed using the unpairedt-test. *P<0.05 (Welch test). (d) Representative FACS analysis. The myeloid progenitors (Lin−IL-7R−Sca-1−c-Kit+) prepared from fetal liver cells of the indicated genotype mice at E11.5 were subfractionated into presumptive common myeloid progenitors (CD34highFcγRII/IIIlow), granulocyte/macrophage progenitors (CD34highFcγRII/IIIhigh) and megakaryocyte/erythroid progenitors (CD34lowFcγRII/IIIlow) by FACS. Axes mean log10fluorescent intensity. (e) TUNEL staining of fetal livers ofUba5+/−andUba5−/−mice at E12.5. Scale bars: top panel, 100 μm; bottom panel, 20 μm. (f) Quantification of mRNA levels of erythroid-related genes, includingGata1,Fog1andEPO,inUba5-deficient liver at E11.5. Total RNAs were prepared from wild-type orUba5-deficient livers and reverse transcribed into their respective cDNAs, which were used as templates for quantitative real-time PCR. Values were expressed relative to the amount of the respective mRNA in the wild-type livers. The experiments were conducted three times. Data are means±s.d. of three experiments. Statistical analysis was carried out by the unpairedt-test. *P<0.05 and **P<0.01 (Welch test). Figure 2: Uba5 is indispensable for the development of erythroid cells. ( a ) Representative FACS analysis. Mouse fetal liver cells were freshly isolated from E11.5 embryos and labelled with a FITC-conjugated anti-CD71 monoclonal antibody and PE-conjugated anti-Ter119 antibody. Left gate : proerythroblast population (Ter119 med CD71 high ), right gate : basoerythroblast population (Ter119 high CD71 high ). Axes mean log 10 fluorescent intensity. ( b ) Quantification of erythroid colony-forming units (CFU-Es) and ( c ) erythroid burst-forming units (BFU-Es). Colony assays were carried out with cells prepared from fetal liver at E11.5. Uba5 deletion was associated with decreased erythroid progenitor activity. Data are means±s.d. of five mice from each group. Statistical analysis was performed using the unpaired t -test. * P <0.05 (Welch test). ( d ) Representative FACS analysis. The myeloid progenitors (Lin − IL-7R − Sca-1 − c-Kit + ) prepared from fetal liver cells of the indicated genotype mice at E11.5 were subfractionated into presumptive common myeloid progenitors (CD34 high FcγRII/III low ), granulocyte/macrophage progenitors (CD34 high FcγRII/III high ) and megakaryocyte/erythroid progenitors (CD34 low FcγRII/III low ) by FACS. Axes mean log 10 fluorescent intensity. ( e ) TUNEL staining of fetal livers of Uba5 +/− and Uba5 −/− mice at E12.5. Scale bars: top panel, 100 μm; bottom panel, 20 μm. ( f ) Quantification of mRNA levels of erythroid-related genes, including Gata1 , Fog1 and EPO, in Uba5- deficient liver at E11.5. Total RNAs were prepared from wild-type or Uba5- deficient livers and reverse transcribed into their respective cDNAs, which were used as templates for quantitative real-time PCR. Values were expressed relative to the amount of the respective mRNA in the wild-type livers. The experiments were conducted three times. Data are means±s.d. of three experiments. Statistical analysis was carried out by the unpaired t -test. * P <0.05 and ** P <0.01 (Welch test). Full size image Each type of common myeloid progenitors (CMPs), granulocyte/macrophage progenitors (GMPs) and megakaryocyte/erythroid progenitors (MEPs) in the bone marrow of adult mice can be distinguished on the basis of the expression of surface markers [21] ( Supplementary Fig. S3c ). In the Lin − IL-7R − Sca-1 − c-Kit + fraction, the CD34 high FcγRII/III low , CD34 high FcγRII/III high and CD34 low FcγRII/III low populations correspond to CMPs, GMPs and MEPs, respectively [21] . To determine whether Uba5 deficiency affects the differentiation steps of these progenitors upstream of BFU-Es and megakaryocytes, the above method was applied to analyse progenitors in Uba5- deficient embryos. As shown in Figure 2d , there was no decrease in the proportion of CD34 high FcγRII/III high (GMPs) populations among the different genotype livers (23.3±2.1% versus 25.4±4.8%, n =3), and the proportion of CD34 high FcγRII/III low (CMPs) was increased in Uba5 -deficient fetal livers (46.0±1.2% versus 59.6±2.3%, n =3, P <0.05). In contrast, the proportion of CD34 low FcγRII/III low population (MEPs) was lower in Uba5 −/− fetal livers (17.1±0.750% versus 4.1±3.5%, n =3, P< 0.05). These results suggest that Uba5 is indispensable for the development of MEPs, but not of GMPs, from CMPs. Loss of Uba5 is accompanied by cell death The total number of fetal liver cells in Uba5 -deficient embryos was significantly lower than in wild-type embryos ( Fig. 1c ). This reduction implies massive loss of erythroid progenitors in Uba5 -deficient fetal livers. Indeed, terminal deoxynucleotidyl transferase (TdT)-mediated dUTP-biotin nick-end labelling (TUNEL) staining showed a significant increase in apoptosis in Uba5- deficient fetal livers at E12.5 ( Fig. 2e ). Quantitative real-time PCR analysis showed underexpression of genes that are specifically expressed in erythroid progenitors, such as Gata1 , Fog1 , β-globin and EpoR (erythropoietin receptor), in Uba5 -deficient fetal livers ( Fig. 2f ). The expression of Epo (erythropoietin) mRNA was augmented in mutant fetal livers, probably because of feedback regulation emanating from the inefficient erythropoiesis in Uba5 −/− embryos ( Fig. 2f ). Taken together, these results suggest that, in addition to efficient differentiation of MEPs, Uba5 is essential for the survival of erythroid progenitors. Generation of transgenic mouse lines of Uba5 driven by G1HRD It is plausible that the defective erythropoiesis and megakaryopoiesis due to loss of Uba5 occurs in a cell-autonomous manner because no impairment of Epo expression was noted in mutant fetal livers ( Fig. 2f ). To prove this hypothesis, we generated transgenic (Tg) mice that expressed both Uba5 and GFP cDNAs under the control of the Gata1 gene haematopoietic regulatory domain (G1HRD) [22] ( Supplementary Fig. S4a ). GATA1 has an important role in erythropoiesis and megakaryopoiesis [23] , [24] . Expression of GATA1 driven by G1HRD rescues the mid-gestational embryonic lethality of Gata1 knockdown mutant mice (Gata1.05) (ref. 25 ). Among several Tg lines, Uba5 #90 exhibited the highest expression of Uba5 in the spleen and bone marrow ( Supplementary Fig. S4b ). In addition, peripheral blood cells from Uba5 #90 mice were positive for GFP, a surrogate marker for the transgene ( Supplementary Fig. S4c ). To further verify that the Uba5 transgene was driven by G1HRD, we examined the lineage of GFP-expressing cells. In Uba5 #90 Tg mice, the majority of GFP-positive cells were found in erythroid ( Supplementary Fig. S4d ) or megakaryocytic ( Supplementary Fig. S4e ) lineages. In contrast, GFP-positive cells were hardly detected in lymphoid (T cells: CD3 + , B cells: B220 + ; see Supplementary Fig. S4f ) and myeloid (Gr1 + Mac1 + , see Supplementary Fig. S4g ) lineages. These results indicate that the expression of Uba5 in the Uba5 #90 line reflects that of the endogenous Gata1 gene, implying that artificial Uba5 is produced in erythroid and megakaryocytic lineages. Therefore, we used the Uba5 #90 line in this study. Cell-autonomous impairment of erythropoiesis in Uba5 −/− mice Uba5 +/− mice were crossed with G1HRD- Uba5 transgenic mice to generate mice that expressed Uba5 in the erythroid lineage ( Uba5 −/− ;Tg Uba5 , hereafter referred to as Uba5 -rescue mice). All Uba5 -rescue mouse embryos were alive at E13.5, in contrast to the death in utero of Uba5 -deficient embryos at the same stage ( Table 2 ), and were morphologically indistinguishable from control mice ( Fig. 3a ). However, the rescue mouse embryos appeared smaller than their control littermates at E15.5 and died by E18.5 ( Fig. 3a and Table 2 ). Importantly, the hypoplasia observed in Uba5 -deficient fetal livers (see Fig. 1a,b ) was significantly ameliorated by the specific expression of Uba5 in the erythroid lineage ( Fig. 3a,b and Supplementary Fig. S5a ). The abnormal multinucleated erythrocytes that were detected in the fetal liver or peripheral blood of Uba5 −/− embryos were not observed in the rescue embryos ( Fig. 3b,d and Supplementary Fig. S5a ). Table 2 Genotypes of embryos obtained from mating Uba5 +/− with Uba5 +/− ;Tg Uba5 mice. 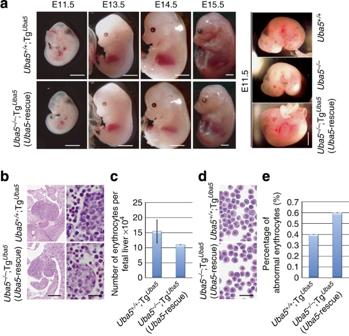Figure 3: Correction of anaemia inUba5-deficient mice by expression ofUba5in erythroid lineage. (a) Embryonic morphology ofUba5rescue mice. Representative photographs ofUba5+/+;TgUba5andUba5−/−;TgUba5embryos at various embryonic stages. Scale bar, 2 mm. (b) Haematoxylin and eosin-stained fetal liver sections ofUba5+/+;TgUba5andUba5−/−;TgUba5mice at E11.5. Scale bars: left panel, 1 mm; right panel, 20 μm. (c) Number of erythroid cells in fetal livers ofUba5+/+;TgUba5andUba5−/−;TgUba5mice at E11.5. Data are means±s.d. of five mice from each group. (d) Wright–Giemsa-stained samples of peripheral blood cytospin cells prepared from control and rescued mice at E11.5. Scale bar, 20 μm. (e) Percentage of abnormal erythrocytes shown ind. Data are means±s.d. of five mice in each group. Full size table Figure 3: Correction of anaemia in Uba5 -deficient mice by expression of Uba5 in erythroid lineage. ( a ) Embryonic morphology of Uba5 rescue mice. Representative photographs of Uba5 +/+ ;Tg Uba5 and Uba5 −/− ;Tg Uba5 embryos at various embryonic stages. Scale bar, 2 mm. ( b ) Haematoxylin and eosin-stained fetal liver sections of Uba5 +/+ ;Tg Uba5 and Uba5 −/− ;Tg Uba5 mice at E11.5. Scale bars: left panel, 1 mm; right panel, 20 μm. ( c ) Number of erythroid cells in fetal livers of Uba5 +/+ ;Tg Uba5 and Uba5 −/− ;Tg Uba5 mice at E11.5. Data are means±s.d. of five mice from each group. ( d ) Wright–Giemsa-stained samples of peripheral blood cytospin cells prepared from control and rescued mice at E11.5. Scale bar, 20 μm. ( e ) Percentage of abnormal erythrocytes shown in d . Data are means±s.d. of five mice in each group. Full size image Next, we examined the effect of Uba5 expression in the erythroid lineage on the differentiation of proerythroblasts and basophilic erythroblasts in Uba5 −/− mice. The decreased population of proerythroblasts and basophilic erythroblasts in Uba5- deficient fetal liver (4.2±3.2% and 1.0±0.6%, respectively, n =3, Fig. 2a ) was rescued by forced expression of Uba5 (9.7±1.6% and 18.2±8.7%, respectively, n =3, Fig. 4a ). Subsequently, we confirmed both CFU-E and BFU-E activities in cells derived from Uba5 -rescued mouse fetal livers ( Fig. 4b,c , and compare with Fig. 2b,c ) as well as the sufficient ability to form CFU-Megs ( Fig. 4d ). As expected, the decreased population of MEPs in Uba5 -deficient fetal liver (4.1±3.5%, n =3, Fig. 2d ) was recovered in the rescued fetal liver (10.2±1.6%, n =3, Fig. 4e ). Moreover, unlike the increase in TUNEL-positive cells in Uba5 -deficient fetal livers, this phenomenon was hardly detected in the rescued mouse livers ( Fig. 4f and Supplementary Fig. S5b ). Taken together, these results indicate that Uba5 expression in erythroid and megakaryocytic progenitors grants functional rescue of defective erythropoiesis and megakaryopoiesis in Uba 5 −/− mice. 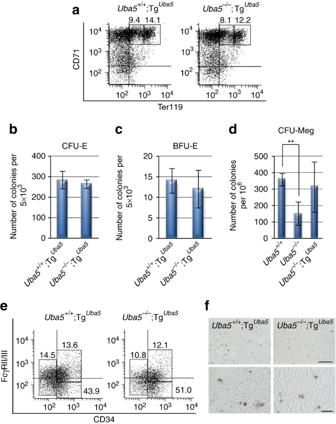Figure 4: Suppression of defective differentiation of both erythrocytes and megakaryocytes following expression of Uba5 in erythroid lineage. (a) FACS analysis. Mouse fetal liver cells were freshly isolated from control and rescued mice at E11.5 and labelled with an FITC-conjugated anti-CD71 monoclonal antibody and PE-conjugated anti-Ter119 antibody.Left gate:proerythroblast population (Ter119medCD71high),right gate:basoerythroblast population (Ter119highCD71high). Axes mean log10fluorescent intensity. (b) Quantification of erythroid colony-forming units (CFU-Es) and (c) erythroid burst-forming units (BFU-Es). Colony assays were carried out with cells prepared from control and rescued fetal liver at E11.5. The number of CFU-E (b) and BFU-E (c) colonies remained unchanged in both genotypes. Data are means±s.d. of five mice from each group. (d) Colony formation assay for megakaryocytes (CFU-Meg). The assays were carried out with cells prepared from the fetal liver of the indicated genotypes at E11.5.Uba5deletion was accompanied by a weaker megakaryocytic differentiation activity, and this defect was suppressed by forced expression of Uba5 in megakaryocytic lineage. Data are means±s.d. ofUba5+/−(n=3),Uba5−/−(n=4) andUba5−/−;TgUba5(n=3). Statistical analysis was carried out using the unpairedt-test. **P<0.01 (Welch test). (e) FACS analysis. The myeloid progenitors (Lin−IL-7R−Sca-1−c-Kit+) prepared from liver cells of control and rescued fetuses at E11.5 were subfractionated into presumptive common myeloid progenitors (CD34highFcγRII/IIIlow), granulocyte/macrophage progenitors (CD34highFcγRII/IIIhigh) and megakaryocyte/erythroid progenitors (CD34lowFcγRII/IIIlow) by FACS. Axes mean log10fluorescent intensity. (f) TUNEL staining of the fetal livers of control and rescue mice at E12.5. Scale bars: top panel, 100 μm; bottom panel, 20 μm. Figure 4: Suppression of defective differentiation of both erythrocytes and megakaryocytes following expression of Uba5 in erythroid lineage. ( a ) FACS analysis. Mouse fetal liver cells were freshly isolated from control and rescued mice at E11.5 and labelled with an FITC-conjugated anti-CD71 monoclonal antibody and PE-conjugated anti-Ter119 antibody. Left gate: proerythroblast population (Ter119 med CD71 high ), right gate: basoerythroblast population (Ter119 high CD71 high ). Axes mean log 10 fluorescent intensity. ( b ) Quantification of erythroid colony-forming units (CFU-Es) and ( c ) erythroid burst-forming units (BFU-Es). Colony assays were carried out with cells prepared from control and rescued fetal liver at E11.5. The number of CFU-E ( b ) and BFU-E ( c ) colonies remained unchanged in both genotypes. Data are means±s.d. of five mice from each group. ( d ) Colony formation assay for megakaryocytes (CFU-Meg). The assays were carried out with cells prepared from the fetal liver of the indicated genotypes at E11.5. Uba5 deletion was accompanied by a weaker megakaryocytic differentiation activity, and this defect was suppressed by forced expression of Uba5 in megakaryocytic lineage. Data are means±s.d. of Uba5 +/− ( n =3), Uba5 −/− ( n =4) and Uba5 −/− ;Tg Uba5 ( n =3). Statistical analysis was carried out using the unpaired t -test. ** P <0.01 (Welch test). ( e ) FACS analysis. The myeloid progenitors (Lin − IL-7R − Sca-1 − c-Kit + ) prepared from liver cells of control and rescued fetuses at E11.5 were subfractionated into presumptive common myeloid progenitors (CD34 high FcγRII/III low ), granulocyte/macrophage progenitors (CD34 high FcγRII/III high ) and megakaryocyte/erythroid progenitors (CD34 low FcγRII/III low ) by FACS. Axes mean log 10 fluorescent intensity. ( f ) TUNEL staining of the fetal livers of control and rescue mice at E12.5. Scale bars: top panel, 100 μm; bottom panel, 20 μm. Full size image In this report, we demonstrated both the specificity of Uba5 for Ufm1 activation and the necessity of the enzyme in erythroid differentiation, suggesting the essential role of one of the ubiquitin-like modification systems, the Ufm1 system, in haematopoiesis and megakaryopoiesis. The most characteristic feature of Uba5 -deficient erythroblasts was the involvement of the multistep process of erythroid differentiation. For instance, despite the insufficient differentiation of MEPs in mutant mice ( Fig. 2d ), partial retention of CFU-E and BFU-E activities was evident ( Fig. 2b,c ), implying that Uba5 -deficient cells that overcome the differentiation step of MEPs can differentiate into mature cells. However, mutant erythroid cells eventually became multinucleated and exhibited an abnormal morphology ( Fig. 1b,f ). Such abnormalities throughout the multistage process were never observed in knockout mice for transcription factors and cytokine receptors that regulate erythroid differentiation, such as the GATA family and EPO-R [23] , [24] , [25] , [26] . The initiation of each step in erythroid differentiation is controlled by the combination of expression of various transcription factors and signal transducers activated by specific cytokines [5] , [6] . Thus, it is plausible that the Ufm1 system modulates the expression levels and/or activation of erythropoiesis-supporting transcription factors. Identification of Ufm1 target(s) is necessary to elucidate how protein modification by Ufm1 regulates erythroid development. In addition, as the volume of circulating primitive erythrocytes in the yolk sac was reduced ( Fig. 1e ) and because such primitive erythrocytes were multinucleated and also showed an abnormal morphology ( Fig. 1d,f ), it is apparent that impairment of both primitive and definitive erythropoiesis is the main cause of death in utero of Uba5 -knockout mice before E13.5 ( Table 1 ). However, in contrast to the almost complete blockade of definitive erythroid differentiation in mutant embryos, the expression of ɛ-globin in the fetal liver was similar to that in control fetal liver ( Fig. 2f ), suggesting a relatively mild defect in primitive erythropoiesis. Thus, we assume that Uba5 deficiency has different effects on primitive and definitive erythropoiesis. Meanwhile, it is obvious that Uba5 is indispensable for the later stage of development because Uba5 -rescued mice did not survive in spite of the marked improvement in Uba5 -based defective erythropoiesis and megakaryopoiesis ( Figs 3 and 4 ). The cause of death might be because of the severe liver hypoplasia that was evident in rescued embryos compared with the control embryos ( Fig. 3a ). The field of haematopoiesis has witnessed tremendous progress in the past decade, specifically in delineating the interplay between lineage-specific cytokines and transcription factors and uncovering the kaleidoscopic pathways of erythrocyte biogenesis in mice [5] , [6] . The present results emphasized the importance of Uba5 in the development of MEPs from CMPs. They also demonstrated that the expression of Uba5 in the erythroid lineage is sufficient for rescuing Uba5 −/− mouse embryos from severe anaemia. Although we cannot exclude other possible function(s) for Uba5 distinct from protein conjugation, as is known for Uba4, the E1 enzyme of the Urm1 system [3] , the results highlight the critical role of the Ufm1 system in the cell-autonomous differentiation process of erythroid progenitors. Generation of Uba5- knockout mice The Uba5 gene was isolated from a mouse B6/C57BL BAC library (MHS1011-58540, Open Biosystems) by hybridization screening. The Uba5 targeting vector was constructed by inserting the neomycin resistance gene instead of the segment that encodes the conserved active-site cysteine residue (Cys250) necessary for activation of Ufm1 ( Supplementary Fig. S2a ). The targeting vector was electroporated into mouse TT 2 ES cells, selected with G418 (250 μg ml −1 ; Invitrogen), and then screened for homologous recombinants by Southern blot analysis. Southern blot analysis was performed by digesting genomic DNA with Spe I (TAKARA BIO) and hybridization to detect 7-kbp and 4-kbp bands that correspond to the wild-type and mutant alleles, respectively. Genotyping of mice was performed by PCR using three primers: 543Fw 5′-CAACTTTGAAGCTCGAATGG-3′, Exon7Rv 5′-CATCCATGTCTGACCAAGTT-3′ and Neopr2 5′-GAAGGGACTGGCTGCTATTGGGCGAAGTGC-3′. Generation of transgenic mice Each Uba5 - and GFP -cDNA was subcloned into the G1HRD vector [25] . The resultant constructs, G1HRD- Uba 5 and G1HRD- GFP , were linearized, and the purified DNAs were co-microinjected into fertilized BDF1 eggs according to standard procedures. Founders were screened by PCR using the following primer sets: for Uba5, the above-described 543Fw and 867Rv 5′-TCATGAACATGGTAGGGAAA-3′, and for GFP, GFP-Fw 5′-AGCAAGGGCGAGGAGCTGTTCACC-3′ and GFP-Rv 5′-TGCCGTCGTCCTTGAAGAAGATG-3′. Uba5 - and GFP -double positive mice were analysed. All experiments involving animals described in the present study were approved by the Animal Ethics Review Committee of the Tokyo Metropolitan Institute of Medical Science. Cell culture and transfection The media and reagents for cell culture were purchased from Life Technologies. HEK293T and MEFs were grown in DMEM containing 10% FCS, 5 U ml −1 penicillin and 50 μg ml −1 streptomycin. HEK293T cells at subconfluence were transfected with the indicated plasmids using Fugene 6 reagent (Roche Molecular Biochemicals). Uba5 +/+ and Uba5 −/− MEFs prepared from 10.5-day embryos were transfected with pMESVts vector, an SV40 large T-antigen expression vector, to establish immortalized MEFs [14] . The immortalized cells were further transfected with the indicated plasmids using the Neon Transfection System (Invitrogen). Cells were analysed at 24 h after transfection. Immunological analysis For immunoblot analysis, cells were lysed with ice-cold TNE buffer (10-mM Tris-Cl, pH 7.5, 1% Nonidet P-40, 150-mM NaCl, 1-mM EDTA and protease inhibitors), and the lysates were separated by the NuPage system (Invitrogen) with 12% bis-tris gels and MOPS-SDS buffer and transferred to a polyvinylidene difluoride membrane. Mouse monoclonal anti-FLAG antibody (M2; Sigma Chemical), Anti-actin antibody (MAB1501R; Chemicon International), Rabbit polyclonal anti-GFP antibody (A6455; Invitrogen), anti-Uba5 antibody [12] and anti-Ufm1 antibody [12] were used for immunodetection. Development was carried out with the Western lighting detection kit (PerkinElmer). The primary antibodies were diluted in the ratio 1:500 with 0.01-M Tris-buffered saline (150 mM NaCl) containing 0.025% Tween-20. For immunoprecipitation analysis, cells were lysed using 200 μl of TNE, and the lysate was then centrifuged at 10,000× g for 10 min at 4 °C to remove debris. Further, 800 μl of TNE and 10 μl of Anti-FLAG M2 agarose affinity gel (Sigma Chemical) or Agarose-conjugated anti-GFP (MBL) were added to the lysate, and the mixture was mixed under constant rotation for 12 h at 4 °C. The immunoprecipitates were washed five times with ice-cold TNE. The complex was boiled for 10 min in SDS sample buffer in the presence of β-mercaptoethanol to elute proteins and centrifuged at 10,000× g for 5 min. The supernatant was subjected to SDS–polyacrylamide gel electrophoresis, transferred to a polyvinylidene difluoride membrane and analysed by immunoblotting with Anti-GFP antibody (A6455; Invitrogen), anti-Ufm1 antibody [12] or anti-Uba5 antibody [12] . Histological examination Embryos in utero were dissected at various stages of development and then fixed in 4% Paraformaldehyde (Nacalai Tesque), paraffin-embedded and sectioned. Paraffin sections were stained with Meyer's haematoxylin and eosin. Apoptotic cells were detected by TUNEL assay [27] . Briefly, cryosections were pretreated with 20 μg ml −1 proteinase K at room temperature for 15 min and then incubated with 100-U ml −1 TdT and 10-nmol ml −1 biotinylated 16-2′-dUTP in TdT buffer (100-mM sodium cacodylatye, pH 7.0, 1-mM cobalt chloride, 50-μg ml −1 gelatin) at 37 °C for 60 min. They were further incubated with peroxidase-conjugated streptavidin for a conventional diaminobenzidine stain. Peripheral blood obtained from embryos was stained with Wright Stain Solution (Wako Pure Chemical Industries) and then with Giemsa Stain Solution (Wako Pure Chemical Industries). Flow cytometry Single cell suspensions were prepared from livers of embryos at E11.5. The cells were incubated in PBS containing 2% fetal bovine serum (FBS; Sigma Chemical) and 2.5-μg ml −1 Fc-block (CD16/CD32, 2.4G2, BD Pharmingen) for 15 min on ice and then stained with antibodies for 20 min on ice. Antibodies for Biotin-CD4 (H129.19), CD8 (53-6.7), B220 (RA3-6B2), Gr-1 (RB6-8C5), Ter119 (TER119), FITC (Fluorescein isothiocyanate)-CD71 (C2), PE (phycoerythrin)-Ter119 (TER119), biotin-Sca-1 (E13-161.7), biotin-IL7R (B12-1), FITC-c-Kit (2B8), PE-FcγRII/III (2.4G2), PE-CD61 (2C9.G2), PE-B220 (RA-6B2), APC-CD3 (17A2), PE-Gr1 (RB6-8C5) and APC-Mac1 (M1/70) were purchased from BD Pharmingen. Streptavidin-ECD (Beckman Coulter) was used as the secondary antibody for biotin. APC (allophycocyanin)-CD34 (RAM34) was purchased from e-Bioscience. The samples were analysed using a FACSCanto II Flow Cytometer (Becton Dickinson). The data were analysed with the Diva 5.0 program (Becton Dickinson). The experiments were conducted three times independently, and their reproducibility was confirmed. Colony assays For the CFU-E assay, 5,000 fetal liver cells were plated in 1 ml of Serum-free methylcellulose (M3234, Stem Cell Technology) supplemented with 10% FBS (Sigma Chemical), 4 U ml −1 Human erythropoietin (Chugai Pharmaceutical) and IMDM. For the BFU-E assay, 5,000 fetal liver cells were plated in 1 ml of serum-free methylcellulose supplemented with 10% FBS (Sigma Chemical), 4 U ml −1 Human erythropoietin (Chugai Pharmaceutical), IMDM and 100-ng ml −1 rmSCF (Kyowa Hakko Kirin). For the CFU-Meg assay, fetal liver cells were cultured with MegaCult-C Kit (Stem Cell Technology) in the presence of 5-ng ml −1 thrombopoietin. Colonies were maintained at 37 °C under humidification and 5% CO 2 . Colonies were scored on day 3 (CFU-E) and on day 7 (BFU-E) by staining with benzidine dihydrochloride. On day 8, clusters containing >10 megakaryocytes were counted as CFU-Meg, on the basis of the manufacturer's instructions. Quantitative real-time PCR Using a Transcriptor First Strand cDNA Synthesis Kit (Roche Applied Science), cDNA was synthesized from 1 μg of total RNA. Quantitative PCR was performed using LightCycler 480 Probes Master (Roche Applied Science) in a LightCycler 480 (Roche Applied Science). Signals were assessed relative to that of β-glucuronidase (GUS). The sequences of the primers used were Gata1 Fw, 5′-GAATCCTCTGCATCAACAAGC-3′; Gata1 Rv, 5′-GGGCAAGGGTTCTGAGGT-3′; Fog1Fw, 5′-AGGCCCCAGGATGAAGAG-3′; Fog1Rv, 5′-ATCCTGCAGTGCCAGCTC-3′; ɛ-GlobinFw, 5′-GATGGAAAAAGATCCAAGCAA-3′; ɛ-GlobinRv, 5′-CACTGTAGCAAGCCGATTTTT-3′; β-GlobinFw, 5′-GGAAAGGTGAACTCCGATGA-3′; β-GlobinRv, 5′-TGGGTCCAAGGGTAGACAAC-3′; EpoFw, 5′-TCTGCGACAGTCGAGTTCTG-3′; EpoRv, 5′-CTTCTGCACAACCCATCGT-3′; EpoRFw, 5′-CCTCATCTCGTTGTTGCTGA-3′; EpoRRv, 5′-CAGGCCAGATCTTCTGCTG-3′; GusFw, 5′-CTCTGGTGGCCTTACCTGA-3′; and GusRv, 5′-CTCAGTTGTTGTCACCTTCACC-3′. Reverse transcription–PCR analysis cDNA was synthesized from 5 μg of DNase I-treated total RNA using the SuperScript First-Strand Synthesis System (Invitrogen) and oligo (dT ) 12–18 primers. The specific primers were 5′-GTGGATTAGAAGAAGGACAAC-3′ and 5′- TCATGAACATGGTAGGGAAA-3′ for Uba5, and 5′-GAGCTGAACGGGAAGCTCAC-3′ and 5′-ACCACCCTGTTGCTGTAGC-3′ for GAPDH. Statistical analysis Statistical analysis was carried out using the unpaired t -test (Welch test) equipped with Excel 2008. Values are means±s.d. For all graphs, data are presented as means±s.d. A P- value <0.05 denoted statistical significance. How to cite this article: Tatsumi, K. et al . The Ufm1-activating enzyme Uba5 is indispensable for erythroid differentiation in mice. Nat. Commun. 2:181 doi: 10.1038/ncomms1182 (2011).